A flow-microreactor approach to protecting-group-free synthesis using organolithium compounds Protecting-group-free synthesis has received significant recent research interest in the context of ideal synthesis and green sustainable chemistry. In general, organolithium species react with ketones very rapidly, and therefore ketone carbonyl groups should be protected before an organolithium reaction, if they are not involved in the desired transformation. If organolithium chemistry could be free from such a limitation, its power would be greatly enhanced. Here we show that a flow microreactor enables such protecting-group-free organolithium reactions by greatly reducing the residence time (0.003 s or less). Aryllithium species bearing ketone carbonyl groups are generated by iodine–lithium exchange reactions of the corresponding aryl iodides with mesityllithium and are reacted with various electrophiles using a flow-microreactor system. The present method has been successfully applied to the formal synthesis of Pauciflorol F. Continuous-flow microreactors based on microfluidics [1] , [2] , [3] have been recognized as powerful tools for chemical synthesis, and studies on their characteristic features have uncovered a rich variety of synthetic applications in recent years [4] , [5] , [6] , [7] , [8] , [9] , [10] , [11] , [12] , [13] , [14] , [15] , [16] , [17] , [18] , [19] , [20] , [21] , [22] , [23] , [24] , [25] . Flow-microreactor synthesis has also received much attention from the viewpoint of synthesis based on reaction integration [26] , [27] , [28] , [29] , [30] and green sustainable synthesis [31] . Such successful applications speak well for the power of the flow-microreactor method in chemical synthesis. It is important to note that the reaction time in a flow microreactor is defined as the residence time between a reagent inlet and the quencher inlet, which can be controlled precisely and reduced to millisecond order by adjusting the length between these positions and the flow speed. On the basis of such a feature of flow microreactors, we have recently proposed the concept of flash chemistry [32] , [33] , [34] , [35] , which enables the use of short-lived highly reactive intermediates for synthesis. Such intermediates can be rapidly generated and transferred to another location in the flow system for use in subsequent reactions before they decompose. It is also noteworthy that the total production capacity over time of continuous-flow microreactors is much greater than may be imagined, although the reactor's capacity at any one time is small. Therefore, flow-microreactor synthesis can be used not only for laboratory-scale synthesis but also for the production of chemical substances on an industrial scale. In fact, there are flow microreactors that fit in the palm of the hand and can produce several tons of products per year [36] , [37] . Armed with an understanding of the essential principles, chemists are now in a position to enhance the capability of flow microreactions and to develop new synthetic transformations that are difficult to achieve by conventional batch reactions. Organolithium species [38] , [39] serve as powerful reagents in organic synthesis. However, they are not compatible with electrophilic functional groups such as ketone carbonyl groups. In fact, organolithium species react with ketones very rapidly. In some cases, organolithium species can be generated in the presence of ketones and quenched in situ by the ketone carbonyl group [40] . However, if a ketone carbonyl group is not involved in the desired transformation, it should be protected before an organolithium reaction, although ketone carbonyl groups survive in reactions of some less reactive organometallics [41] , [42] , [43] . Therefore, if organolithium reactions can be conducted without protecting the ketone carbonyl groups, the power of organolithium chemistry will be greatly enhanced. Here we show that a flow microreactor enables protecting-group-free organolithium reactions by greatly reducing the residence time (0.003 s or less); aryllithium species bearing ketone carbonyl groups are generated by iodine–lithium exchange reactions of the corresponding aryl iodides with mesityllithium and are reacted with various electrophiles using a flow-microreactor system by greatly reducing the residence time (0.003 s or less). We also show that the present method has been successfully applied to the formal synthesis of Pauciflorol F. 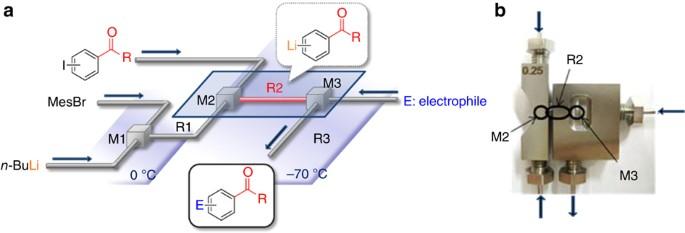Figure 1: A flow-microreactor system. (a) A schematic diagram of the system. 2-Bromo-1,3,5-trimethylbenzene (mesityl bromide, MesBr) was reacted withn-butyllithium using T-shaped micromixer M1 and microtube reactor R1 at 0 °C. The resulting mesityllithium solution was reacted with an acyliodobenzene in T-shaped micromixer M2 and microtube reactor R2 at −70 °C. The resulting short-lived acylphenyllithium species was trapped with an electrophile using T-shaped micromixer M3 and microtube reactor R3 at −70 °C. (b) An integrated device in which M2 (inner diameter: 250 μm), R2 (inner diameter: 250 μm, length: 1.0 cm) and M3 (inner diameter: 250 μm) are combined. Generation and reactions of acyl-substituted aryllithiums We began our investigation by conducting the iodine–lithium exchange reaction of o - and p -acyliodobenzenes followed by trapping with methanol using the flow-microreactor system, as shown in Figure 1 (see also Supplementary Fig. S1 ). Mesityllithium was first generated by a bromine–lithium exchange reaction of 2-bromo-1,3,5-trimethylbenzene (mesityl bromide) and n -butyllithium at 0 °C, because preliminary studies showed that mesityllithium was the most effective compound for this purpose. The iodine–lithium exchange reaction of an acyliodobenzene using the resulting mesityllithium was conducted at −70 °C. The short-lived acylphenyllithium species thus produced was trapped with methanol as an electrophile at −70 °C ( Fig. 1a ). Figure 1: A flow-microreactor system. ( a ) A schematic diagram of the system. 2-Bromo-1,3,5-trimethylbenzene (mesityl bromide, MesBr) was reacted with n -butyllithium using T-shaped micromixer M1 and microtube reactor R1 at 0 °C. The resulting mesityllithium solution was reacted with an acyliodobenzene in T-shaped micromixer M2 and microtube reactor R2 at −70 °C. The resulting short-lived acylphenyllithium species was trapped with an electrophile using T-shaped micromixer M3 and microtube reactor R3 at −70 °C. ( b ) An integrated device in which M2 (inner diameter: 250 μm), R2 (inner diameter: 250 μm, length: 1.0 cm) and M3 (inner diameter: 250 μm) are combined. Full size image We focused on the generation of o -pentanoyl-substituted phenyllithium ( 2 ) generated from o -pentanoyliodobenzene ( 1 ). Methanol was used as a quenching electrophile ( Fig. 2a ). The reactions were carried out with variation in the residence time in R2, and the yield of the protonated product 3 was determined by gas chromatography (GC). The yield of 3 increased with a decrease in the residence time ( Fig. 2b , see also Supplementary Table S1 ). However, acceptable yields were not obtained even at the minimum limit of the residence time of our current system (0.01 s), although this residence time was successful for the generation of alkoxycarbonyl- [44] , nitro- [45] and cyano-substituted [46] aryllithiums. Aryllithium 2 bearing a ketone carbonyl group decomposed very rapidly, the major by-product being dimeric compound 4 . 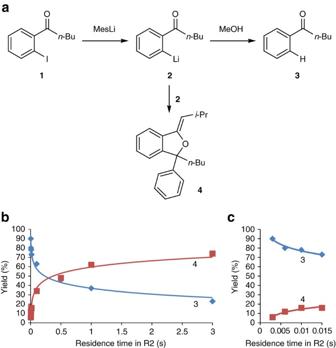Figure 2: The effect of residence time in R2 for the reaction ofo-pentanoyliodobenzene (1). (a) Reaction of1with MesLi to yieldo-pentanoyl-substituted phenyllithium (2) followed by trapping with MeOH to produce protonated product3. Undesired dimerization of2gave by-product4. (b) Plots of the yield of3and4against the residence time in R2 (<3 s). (c) Plots of the yield of3and4against the residence time in R2 (<0.015 s). Figure 2: The effect of residence time in R2 for the reaction of o -pentanoyliodobenzene ( 1 ). ( a ) Reaction of 1 with MesLi to yield o -pentanoyl-substituted phenyllithium ( 2 ) followed by trapping with MeOH to produce protonated product 3 . Undesired dimerization of 2 gave by-product 4 . ( b ) Plots of the yield of 3 and 4 against the residence time in R2 (<3 s). ( c ) Plots of the yield of 3 and 4 against the residence time in R2 (<0.015 s). Full size image To avoid the decomposition of 2 , we developed a new integrated device in which two T-shaped micromixers and one microreactor are combined ( Fig. 1b ). Although the Reynolds number is ∼ 10 2 , extremely fast mixing takes place at the T-shaped mixers, presumably because of engulfment flow [47] . Using this device, the residence time could be reduced to 0.003 s, giving rise to a dramatic increase in the yield of product 3 ( Fig. 2c ). The result clearly indicates that a ketone carbonyl group could survive a residence time of a few milliseconds. At a residence time of 0.003 s, generation of various o -acyl-substituted aryllithium species followed by reactions with various electrophiles including Me 3 SiOTf, Bu 3 SnCl and ClCO 2 Me were successfully conducted, and the corresponding products bearing unchanged ketone carbonyl groups were obtained in good yields and productivity (0.25–0.54 mmol min −1 ; Table 1 , entries 1–12). It is interesting that some ketones could be used as electrophiles, although they should be more reactive than the carbonyl group of the acylphenyllithium species (entries 5 and 6). Table 1 Generation of acyl-substituted aryllithiums and reactions with electrophiles in a flow-microreactor system. Full size table The generation and reaction of p -acyl-substituted phenyllithiums led to slightly lower yields of the products (entries 13–21) compared with the corresponding o -acyl-substituted phenyllithiums, presumably because of the lack of coordination of the carbonyl group to lithium. In particular, in the case of p -acetylphenyllithium ( 6 ) generated from p -acetyliodobenzene ( 5 ), the protonated product 7 was obtained only in moderate yield (54%, entry 20). This problem could be solved by further reducing the residence time in R2, which was achieved by increasing the flow rate using a high-pressure syringe pump. 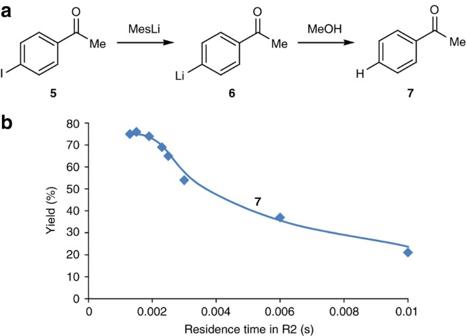Figure 3: The effect of residence time in R2 for the reaction ofp-acetyliodobenzene (5). (a) Reaction of5with MesLi to yieldp-acetylphenyllithium (6) followed by trapping with MeOH to produce protonated product7. (b) Dependence of the yield of7on the residence time in R2 (<0.01 s). As shown in Figure 3 , the yield of 7 increased with a decrease in the residence time, and an acceptable yield (76%) was obtained at a residence time of 0.0015 s (see also Supplementary Table S2 ). This residence time also allowed efficient reaction with PhCHO to produce the corresponding product in 78% yield (entry 21). Heteroaromatic iodides such as 1-(5-iodothiophen-2-yl)pentan-1-one 31 could also be lithiated and the resulting organolithium compounds were effectively trapped with electrophiles without affecting the ketone carbonyl group (entries 22–24). Figure 3: The effect of residence time in R2 for the reaction of p -acetyliodobenzene ( 5 ). ( a ) Reaction of 5 with MesLi to yield p -acetylphenyllithium ( 6 ) followed by trapping with MeOH to produce protonated product 7 . ( b ) Dependence of the yield of 7 on the residence time in R2 (<0.01 s). Full size image Application to formal synthesis of Pauciflorol F Using the present method, Pauciflorol F [48] , a natural product isolated from stem bark, which has recently been synthesized by Snyder's group [49] , [50] and Sarpong's group [51] , was synthesized. The starting material 35 was prepared from commercially available 3,5-dimethoxyphenylmagnesium chloride in two steps (67% yield; Fig. 4 ). The iodine–lithium exchange reaction of 35 followed by reaction with 3,5-dimethoxybenzaldehyde was conducted using a flow-microreactor system consisting of the integrated device (residence time in R2: 0.003 s) to produce 36 (ref. 49 ) in 81% isolated yield. Presumably, dehydration took place upon acidic work-up. Treatment of 36 with HCl/ i -PrOH in the presence of O 2 in a batch reactor gave 37 in 75% yield, which can be converted to Pauciflorol F by one-pot hydrogenation and epimerization (87%) [51] followed by deprotection (86%) [49] , [50] . 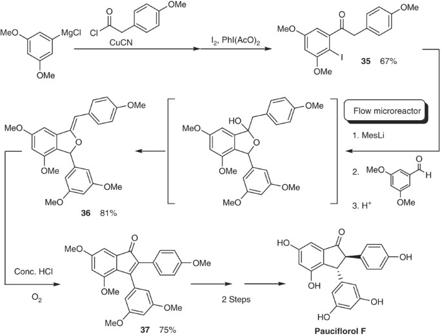Figure 4: Formal total synthesis of Pauciflorol F. The flow-microreactor reaction of iodoketone35gave compound36(81% yield, 1.06 g for 5 min operation), which can be converted to Pauciflorol F according to the literature procedure. Figure 4: Formal total synthesis of Pauciflorol F. The flow-microreactor reaction of iodoketone 35 gave compound 36 (81% yield, 1.06 g for 5 min operation), which can be converted to Pauciflorol F according to the literature procedure. Full size image Recently, the construction of complicated organic molecules without using protecting groups (protecting-group-free synthesis) [52] , [53] , especially from the viewpoints of atom economy [54] , step economy [55] and redox economy [56] , has received significant research interest in the context of ideal synthesis [57] and green sustainable chemistry [58] . Generally, skeleton-building steps are the most difficult with respect to avoiding usage of protecting groups because such steps often use strongly basic nucleophilic reagents. Among such reagents, organolithium reagents are the most reactive. However, a major drawback of organolithium species is that they are too reactive and rapidly react with electrophilic functional groups such as ketone carbonyl groups, which are often present in the desired target organic structures. Therefore, organic textbooks say that a ketone carbonyl group should be protected before an organolithium reaction if it is not involved in the desired transformation. However, we have demonstrated here that aryl- and heteroaryllithium species bearing ketone carbonyl groups can be generated and used for desired reactions by greatly reducing the residence time in a flow microreactor to a few milliseconds. Within such an extremely short residence time, the organolithium intermediates can survive and be used for reactions with various external electrophiles without affecting the ketone carbonyl group in the same molecule. The formal synthesis of Pauciflorol F achieved in this study ( Fig. 4 ) demonstrates the potential of the present flow-microreactor approach. Although the synthesis by Snyder's group based on a biomimetic strategy and the synthesis by Sarpong's group based on a Larock annulations strategy are elegant and concise, our synthesis is comparable from the viewpoints of atom economy and step economy. Because the productivity of the present method is relatively high (1.06 g for 5 min operation), it is hoped that the flow-microreactor method will provide a green and sustainable way of producing useful compounds such as Pauciflorol F in the pharmaceutical and fine chemicals industries in the future. The present approach based on control of the residence time in a flow microreactor serves as a powerful method for protecting-group-free synthesis using organolithium reagents, which is complementary to other approaches using less reactive and more chemoselective reagents. Although the flow-microreactor approach is still in its infancy, it is clearly capable, powerful and useful from both scientific and practical viewpoints. Currently, work to expand further the capability of flow-microreactor synthesis is in progress. General procedure A flow-microreactor system consisting of three T-shaped micromixers (M1, M2 and M3) and three microtube reactors (R1, R2 and R3) was used. A solution of mesityl bromide in tetrahydrofuran (THF; 0.18 M, flow rate: 5.0 ml min −1 ) and a solution of n -BuLi in hexane (0.43 M, flow rate: 1.8 ml min −1 ) were introduced to M1 (inner diameter: 250 μm). The resulting solution was passed through R1 and was mixed with a solution of acyliodobenzene in THF (0.20 M, flow rate: 3.0 ml min −1 ) in M2 (inner diameter: 250 μm). The resulting solution was passed through R2 and then mixed with a solution of an electrophile (0.60 M, flow rate: 2.0 ml min −1 ) in M3 (inner diameter: 250 μm). The resulting solution was passed through R3. After a steady state was reached, the product solution was collected for 30 s while being quenched with aqueous sat. NH 4 Cl solution (2 ml). The aqueous layer was extracted three times with ether (25 ml). The combined organic extracts were dried over Na 2 SO 4 and concentrated. The crude product was purified by chromatography. Details of the synthesis, purification and characterization are given in Supplementary Figures S2–S25 . Formal total synthesis of Pauciflorol F In all, 1 M CuCN·2LiCl THF solution (44 ml, 44.0 mmol) was added dropwise to a solution of 3,5-dimethoxyphenylmagnesium chloride (0.5 M in THF, 80 ml, 40.0 mmol) at −25 °C for 10 min. After being stirred for 40 min at −20 °C, 4-methoxyphenylacetyl chloride (9.793 g, 53.0 mmol) was added dropwise for 5 min. The solution was slowly warmed to −10 °C for 1 h, and the reaction was quenched by slow addition of sat. NH 4 Cl solution (120 ml). The organic layer was separated and the aqueous layer was extracted with Et 2 O (150 ml×3). The combined organic layers were dried over Na 2 SO 4 and concentrated. The crude product was purified by column chromatography (CHCl 3 ) and washed with cold hexane to obtain 1-(3,5-dimethoxyphenyl)-2-(4-methoxyphenyl)ethanone in 91% yield ( Supplementary Fig. S26 ). Iodobenzene diacetate (242.0 mg, 0.75 mmol) was added to a solution of 1-(3,5-dimethoxyphenyl)-2-(4-methoxyphenyl)ethanone (146.8 mg, 0.51 mmol) and iodine (70.9 mg, 0.28 mmol) in CH 2 Cl 2 (4 ml) at 0 °C. After being stirred at 0 °C for 10 h, the solution was slowly warmed to ambient temperature. After being stirred for 14 h, the reaction was quenched by addition of half-saturated Na 2 S 2 O 3 solution (10 ml). The organic layer was separated and the aqueous layer was extracted with CH 2 Cl 2 (25 ml×3). The combined organic layers were dried over Na 2 SO 4 and concentrated. The crude product was purified by column chromatography (hexane/AcOEt=4:1) to obtain 1-(2-iodo-3,5-dimethoxyphenyl)-2-(4-methoxyphenyl)ethanone ( 35 ) in 74% yield ( Supplementary Fig. S27 ). The flow-microreactor system shown in Figure 1a containing the integrated device ( Fig. 1b ) was used. A solution of 2-bromomesitylene (0.18 M in THF, 5.0 ml min −1 ) and a solution of n -BuLi (0.43 M in hexane, 1.8 ml min −1 ) were introduced to M1 (inner diameter: 250 μm) by syringe pumps. The resulting solution was passed through R1 (inner diameter: 1,000 μm, length: 210 cm (100 cm at 0 °C, 10 cm at ambient temperature and 100 cm at −70 °C)) and was subsequently mixed with a solution of acyliodobenzene 35 (0.20 M in THF, 3.0 ml min −1 ) at M2 (inner diameter: 250 μm). The resulting solution was passed through R2 (inner diameter: 250 μm, length: 1.0 cm) and 3,5-dimethoxybenzaldehyde (0.60 M in THF, 2.0 ml min −1 ) was added at M3 (inner diameter: 250 μm). The resulting solution was passed through R3 (inner diameter: 1,000 μm, length: 50 cm). After a steady state was reached, the product solution was collected for 5 min while being quenched with H 2 O (20 ml). After 1 M HCl solution (80 ml) was added, the organic layer was separated and the remaining aqueous layer was extracted with Et 2 O (100 ml×3). The combined organic layers were dried over Na 2 SO 4 and concentrated. The crude product was purified by column chromatography (hexane/AcOEt=2:1) to obtain 3-(3,5-dimethoxyphenyl)-4,6-dimethoxy-1-(4-methoxybenzylidene)-1,3-dihydroisobenzofuran ( 36 ) in 81% yield (1.058 g; Supplementary Fig. S28 ). Aqueous conc. HCl solution (4 ml) was added dropwise for 30 min to a solution of 36 (44.0 mg, 0.101 mmol) in i -PrOH (20 ml) at 25 °C. After being stirred for 12 h under an oxygen atmosphere, the reaction was quenched by slow addition of aqueous sat. NaHCO 3 solution (60 ml) and water (40 ml) at 0 °C. The organic layers were extracted with AcOEt (40 ml×3) and washed with brine (40 ml). The combined organic layers were dried over Na 2 SO 4 and concentrated. The crude product was purified by column chromatography (hexane/AcOEt=3:1) to obtain 3-(3,5-dimethoxyphenyl)-4,6-dimethoxy-2-(4-methoxyphenyl)-1H-inden-1-one ( 37 ) in 75% yield ( Supplementary Fig. S29 ), which can be converted to Pauciflorol F by one-pot hydrogenation and epimerization followed by deprotonation. How to cite this article: Yoshida, J.-i. et al . A flow-microreactor approach to protecting-group-free synthesis using organolithium compounds. Nat. Commun. 2:264 doi: 10.1038/ncomms1264 (2011).